Flow velocities of Alaskan glaciers Our poor understanding of tidewater glacier dynamics remains the primary source of uncertainty in sea level rise projections. On the ice sheets, mass lost from tidewater calving exceeds the amount lost from surface melting. In Alaska, the magnitude of calving mass loss remains unconstrained, yet immense calving losses have been observed. With 20% of the global new-water sea level rise coming from Alaska, partitioning of mass loss sources in Alaska is needed to improve sea level rise projections. Here we present the first regionally comprehensive map of glacier flow velocities in Central Alaska. These data reveal that the majority of the regional downstream flux is constrained to only a few coastal glaciers. We find regional calving losses are 17.1 Gt a −1 , which is equivalent to 36% of the total annual mass change throughout Central Alaska. Mountain glaciers are significant contributors to current and future sea level rise (SLR). Worldwide, mountain glaciers contribute to about half of the new-water SLR from land ice [1] , but the proportion of mass lost due to changing ice flow dynamics is unknown and likely large [1] . In southeastern Alaska and northwest British Columbia, up to 66% of the mass loss may be a consequence of accelerating ice flow and resultant calving into tidewater or lake environments [2] . Elsewhere in Alaska, immense lake and tidewater dynamic mass losses [2] , [3] , [4] , [5] have been observed as well. Such mass losses are a consequence of a positive feedback mechanism that accelerates ice flow and calving rate [6] . This feedback is typically triggered through a reduction in resistive back stress that can come from submarine melting [7] , [8] , changes in front position [9] , [10] , and/or a reduction in ice front mélange concentration [11] . These mechanisms can often lead to seasonal oscillations in iceberg calving with peak calving rates in spring and early summer [7] , [11] . Because of these dynamics, uncertainties in future calving loss projections are very different (and larger) from uncertainties in surface mass balance (SMB) projections. SMB projections are constrained using physically grounded models [12] . However, projections of mountain glacier mass loss that include calving are forced to use simple linear extrapolations because tidewater dynamics are so poorly understood. If we are to reduce uncertainties in SLR projections, partitioning of current mass loss sources will help to constrain projections of calving mass loss and will help to reconcile SMB models and gravimetrically derived total mass balance estimates [13] , [14] . Ice dynamics may also affect mass balance on land-terminating glaciers [15] . Meltwater-induced basal lubrication can cause brief acceleration, particularly in spring [16] , [17] , [18] . Warmer summers have also been shown to cause slower flow in late summer [19] . However, these dynamics are poorly understood; in particular, we lack understanding of how the responsible mechanisms may evolve in a changing climate. In western Greenland and in some mountain glacier areas [20] , [21] , flow velocities have slowed over long periods but elsewhere changes are not known due to a lack of velocity data. Ice dynamics on surge-type glaciers also likely have an impact on mass balance. Surge-type glaciers undergo periodic accelerations of 10–100 times normal velocities [22] , [23] , this dynamic redistributes mass to lower elevations and thus increases SMB mass losses. Surging can also increase ablation rates by exposing greater surface area through crevassing [24] . Given that surge-type glaciers never flow in equilibrium with climate [23] , their dynamic response to climate change and mass loss will likely be different than responses from other glaciers. Alaska has the highest concentration of surge-type glaciers in the world [25] and while the surge cycle has been studied thoroughly on a few glaciers [22] , [23] , [26] , [27] , nearly 200 surge-type glaciers in Alaska are devoid of observation [25] . Therefore, regional observations of velocities on surge-type glaciers, both during surge and quiescent (slow) phases are needed to address regional dynamics on these unique systems. Surging and tidewater related mass loss also has important tectonic implications in the St Elias Mountains by affecting fault stability in areas capable of generating large magnitude earthquakes [28] , [29] . Mapping mountain glacier velocities on regional scales has different impediments than doing so on the ice sheets. Mountain glaciers are often in extremely cloudy, maritime environments that conceal the glacier surface from optical satellites and change surface conditions rapidly. Southern Alaska typifies this environment with up to 5 m.w.e. of snowfall and 12 m.w.e. of melt annually [30] . In these environments, synthetic aperture radar (SAR) satellite platforms have advantages and disadvantages over optical sensors. SAR penetrates cloud cover and is able to track velocities in featureless accumulation zones. SAR interferometry has proven effective on the ice sheets but this method is extremely vulnerable to rain and summertime melt. A more robust method, offset tracking, uses two images acquired at different times to find the horizontal displacement of pixel patterns using cross-correlation [31] , [32] , [33] . Offset tracking is effective using both optical and SAR platforms, and has produced velocity results in many mountain glacier regions [34] , [35] , [36] , [37] , including Alaska [21] . However, assessing ice dynamic SLR contribution from mountain glaciers requires more comprehensive studies. We expand upon this work spatially and target areas that are likely to have large mass losses due to ice dynamics. We processed 344 SAR image pairs and selected the best data, which were acquired between 2007 and 2010, to produce mosaicked velocity maps (see Methods). The velocity maps allow for a rough estimate of regional glacier calving flux for 20 tidewater and 16 lacustrine glacier termini using crude assumptions of ice thickness (see Methods). While the method used is simplified, more sophisticated methods still contain large biases compared with volume/area scaling in Alaska [38] and are otherwise not validated. Limited opportunities to validate our thickness estimates are available on a few glaciers (see Methods). Overall, the maps presented indicate that the majority of the downstream flux is not necessarily linked to tidewater dynamics as for the ice sheets [39] , [40] , rather the majority of the downstream flux is related to exceptionally high accumulation rates on specific glaciers. Such differences will likely lead Alaska glaciers to different dynamic responses to climate change than on the ice sheets. We are also able to derive estimates of current regional calving loss, which offer a first opportunity to partition 47 Gt a −1 of total mass loss throughout the region [13] . Regional calving losses are estimated to be 17 Gt a −1 (and between 18 Gt a −1 and 13 Gt a −1 ), which is equivalent to ~36% of the total annual mass change throughout Central Alaska; thus implying regional SMB net change of 30 Gt a −1 (or between 26 and 34 Gt a −1 ). Surface velocity maps Surface velocities are available for 28,022 km 2 of glacier area, which includes almost all major glaciers in Alaska west of 138 ° W; expanding these data east will follow in later papers. Our uncertainties are quantified using a robust equivalent to a 1-sigma uncertainty and are 0.02 m per day (see Methods section). We derive mosaicked velocity maps for the Wrangell-St. Elias Mountains ( Fig. 1 ), the Chugach Mountains/Kenai Peninsula ( Fig. 2 ), the Alaska Range ( Fig. 3 ) and the Tordrillo Range ( Fig. 4 ). These maps resolve mean velocities over 46-day orbit intervals. Of the 60 image pairs used for the map, 56 were acquired in January and February ( Fig. 5 ). Although annual average velocities would be ideal, shorter repeats allow for less decorrelation and are necessary for the spatial coverage we have achieved. Nonetheless, January/February velocities can still be considered representative of mean annual velocities. Some glaciers in Alaska have shown little to no seasonal variability [41] . Others do have variations, but have been observed to have velocity maximums in spring, minimums in fall and intermediate speeds in mid-winter. This case has been observed both on land-terminating glaciers [19] and tidewater glaciers in Alaska [42] . Wintertime velocities are also the most constant over short time periods [43] and thus the most likely to provide consistency in observations. Still, many glaciers underwent significant inter-annual velocity variability over the observation interval and only one velocity snapshot is included in this map ( Figs 1 , 2 , 3 , 4 ). 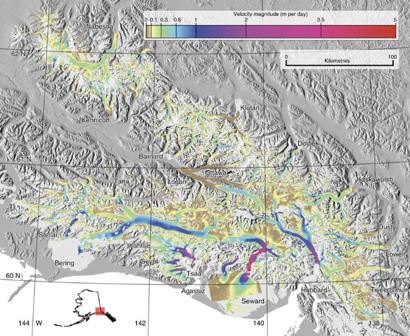Figure 1: Surface velocity map of the Wrangell and St Elias Ranges. Light grey glacier outlines47indicate missing data. Figure 1: Surface velocity map of the Wrangell and St Elias Ranges. Light grey glacier outlines [47] indicate missing data. 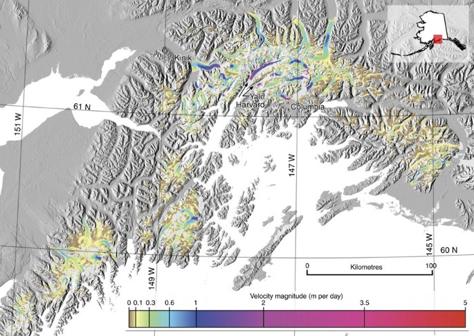Figure 2: Surface velocity map of the Chugach Range and Kenai Peninsula. White glacier outlines47indicate missing data. Full size image Figure 2: Surface velocity map of the Chugach Range and Kenai Peninsula. White glacier outlines [47] indicate missing data. 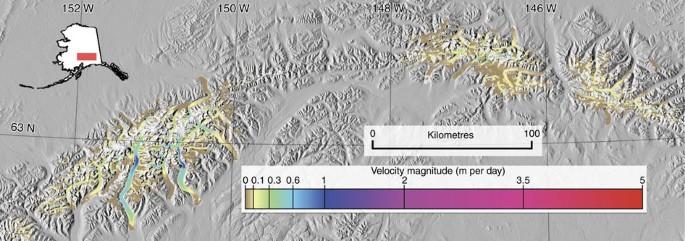Figure 3: Surface velocity map for the Alaska Range. Light grey glacier outlines47indicate missing data. Full size image Figure 3: Surface velocity map for the Alaska Range. Light grey glacier outlines [47] indicate missing data. 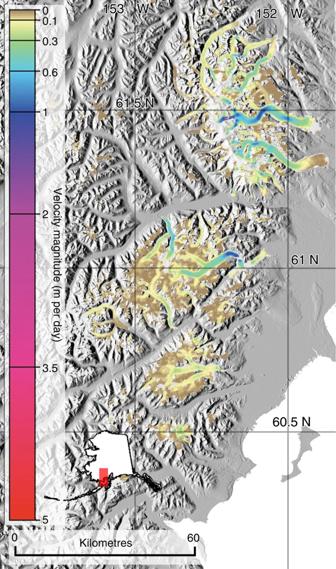Figure 4: Surface velocity map for the Tordrillo Range. Light grey glacier outlines47indicate missing data. Full size image Figure 4: Surface velocity map for the Tordrillo Range. Light grey glacier outlines [47] indicate missing data. 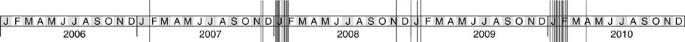Figure 5: Dates of all 60 image pairs composing the velocity maps. Each line represents the mean day between a 46-day acquisition interval. Full size image Figure 5: Dates of all 60 image pairs composing the velocity maps. Each line represents the mean day between a 46-day acquisition interval. Full size image Spatial structure of velocity The regional spatial structure of flow velocity conforms to our understanding of glacier balance velocities (a flow speed that compensates for accumulated mass upstream) and surge dynamics. Flow velocities generally increase from continental climes towards the maritime coast. In particular, there are 12 glacier systems that have exceptionally high velocities (>1 m per day) over much of their length. The fast velocities are not necessarily linked to tidewater dynamics—these twelve glaciers include land-terminating glaciers in addition to calving glaciers in retreat and advance: Hubbard, Seward, Agassiz, Yahtse, Guyot, Tsaa, Stellar, Bering, Columbia, Harvard, Yale and Knik Glaciers. Rather, these 12 glaciers all have high elevation, coastal accumulation zones and are consequently positioned to receive the highest accumulation rates throughout Alaska. Thus, these glaciers would require large fluxes to balance accumulation. We provide a crude estimate of total downstream ice flux by spatially integrating the velocity field within individual glacier basins to obtain a total surface area flux per glacier (units: km 2 m per day). This analysis is not a volumetric flux and does not account for missing data. Nonetheless, we find that Seward, Bering, Hubbard, Yahtse, Guyot and Tsaa Glaciers account for ~50% of the total flux throughout the data set. If data coverage were better, we expect Columbia, Harvard, Yale and Knik would take on similar importance (our patchy results indicate high velocities on these glaciers as well). Surge-type glaciers The velocity maps also include flow speeds on more surge-type glaciers than ever compiled previously. During the observation period (2007–2011), temporal velocity variability was observed on many surge-type glaciers. However, out of 22 large surge-type glaciers, surges (defined as variations in velocity >10 times observed slow values) were only observed on Bering, Lowell and Ottawa ( Fig. 1 ), and only Bering is in surge phase in the maps presented (due to data availability). Given that surge intervals in Alaska are between 18 and 75 years [27] , [44] , we would expect to see somewhere between 11 and 3 surges for maritime and continental climates, respectively. Given that most of the surge-type glaciers are in continental climates, long-term regional mean fluxes from surge-type glaciers are likely underestimated in this map, but not massively. Flow speeds of surge-type glaciers [25] in quiescence are almost always flowing slower than neighbouring glaciers that are not surge-type. Most surge-type glaciers have expansive areas of stagnant ice at their termini and higher velocities upstream. Mapped data on Tweedsmuir Glacier ( Fig. 1 ) immediately follows a surge ending in 2009; these data show stagnant ice throughout the glacier length. These configurations conform well to observations and model results on Variegated Glacier [26] , [45] , suggesting that most surge-type glaciers are undergoing similar quiescent phase evolutions. There are, however, a few notable exceptions ( Fig. 1 ). Quiescent phase velocities on Seward Glacier exceed 5 m per day, which are, by far, the highest land-terminating flow speeds in the data set. How Seward Glacier is able to maintain these velocities during quiescence may be due to its bi-modal elevation distribution. Donjek Glacier (surge-type) also has exceptionally high velocities when compared with neighbouring systems in quiescence. Lowell Glacier surged in 2010 a year prior ice velocities were relatively high near the terminus and slower upstream as shown in Fig. 1 . Calving flux We estimate calving fluxes from 20 tidewater and 16 lacustrine glaciers in Central Alaska to be 9.1 Gt a −1 ( Table 1 ). Uncertainty bounds on this estimate are large, but are difficult to derive due to a paucity of ice thickness data. Therefore, we bracket our flux estimates (see Methods) and find that calving losses from the glaciers considered are unlikely to be higher than 10 Gt a −1 and unlikely to be lower than 5.1 Gt a −1 . These numbers do not include 10 small tidewater glaciers and many small lacustrine glaciers within the study area. These numbers also do not include Columbia Glacier, which is moving too fast for our methods. Discharge from Columbia [46] has been estimated to be 8 Gt a −1 by subtracting modelled SMB from geodetically determined total mass loss. Table 1 Calving fluxes. Full size table If calving loss from Columbia is included [46] , we find the Central Alaska calving loss to be 17.1 Gt a −1 (and between 18 Gt a −1 and 13.1 Gt a −1 ). While, there is no robust estimate of SMB within the same area to provide a comparison, 17.1 Gt a −1 of calving loss is equivalent to 36% of the total annual mass change [13] (−47 Gt a −1 ) throughout the Wrangell/St Elias, Chugach, Kenai, Tordrillo and Alaska Ranges (as determined from GRACE observations [13] ). This implies that if calving were to cease, the rate of total mass loss would drop by 36%; or if calving were to double, total mass loss would increase by 36%. Efficacy of SAR offset tracking in Alaska The only SAR platforms with extensive geographical/temporal coverage are ALOS PALSAR, RADARSAT and ERS-1/2. Of these, only ALOS (L-Band) is robust in Alaska’s maritime environment and effective in featureless accumulation zones. Given the harshness of Alaska’s environment, it is likely that results of similar/improved quality can be obtained on mountain glaciers worldwide. However, none of these platforms are effective in summer because of surficial melting; none are effective at coastal low elevations due to rain; and none are effective on fast moving ice because of long-repeat times. These limitations are problematic as it is these areas that are experiencing the most rapid changes in flow velocities, typically related to tidewater dynamics. Short-repeat platforms, including TerraSAR-X and ERS Tandem/Ice Phase were found to be effective in these environments despite having shorter wavelengths that are more sensitive to water. However, data acquired by these platforms are geographically/temporally limited and have lower precision because of a necessary shorter acquisition interval. The data set presented represents the first regional map of mountain glacier flow speeds in Alaska. The velocity magnitude data will be available for public download at the Alaska Satellite Facility ( http://www.asf.alaska.edu/ ). These maps provide wintertime flow speeds on almost every major glacier system in the Wrangell/St Elias, Chugach, Kenai Peninsula, Alaska and Tordrillo Ranges. We note that inter-annual fluctuations in winter velocity were found on many glaciers between 2007 and 2011. Thus, caution should be used when examining multi-year trends in glacier velocities because assuming uniform multi-year velocity change is not necessarily valid. This variability will be discussed in a later paper. The results presented here are critical because they enable us to place focused studies of dynamics in the broader context of 25,000+ glaciers in Alaska [47] . Many surging glaciers in the data set appear to be undergoing similar quiescent phase velocity evolutions as observed more closely on Variegated Glacier. Other surge-type glaciers appear to be exhibiting other unresolved dynamics. Columbia contributes to 51% of the total calving flux throughout the region. Generally, flow velocities on the southern coast are far higher than areas inland. We find that the ice flux from the 12 fast flowing glaciers mentioned is immense with respect to Alaska as a whole. Given that these glaciers are likely thicker than others (they are significantly larger in area than the average), it is likely that these 12 glaciers account for far more than half of the volumetric flux throughout Alaska. On the ice sheets, anomalously large fluxes are typically the result of outlet glacier retreat [39] , [40] . However in Alaska, extremely large gradients in snow accumulation rates force anomalously high balance velocities on glaciers with high elevation coastal accumulation zones, which happens to include surging glaciers, land-terminating glaciers and lake/tidewater glaciers in retreat and advance. This does not imply that the largest mass losses are coming from these glaciers, but we suggest that dynamics on these rapid-flow systems may operate differently than other glaciers, because they are able to maintain higher flow speeds and higher driving stresses without losing mass. Thus long-term ice dynamic response to climate change in Alaska will likely evolve differently than in areas where outlet glaciers dominate regional downstream fluxes. Understanding the dynamics of these 12 glacier systems is critical for future efforts to estimate dynamic mass loss in Alaska. The key finding from this work is that iceberg calving currently contributes −17 Gt a −1 (or between 18 Gt a −1 and 13 Gt a −1 ) to the mass budget in Alaska. This number is equivalent to 36% of the total annual mass change throughout the Wrangell/St Elias, Chugach, Kenai, Tordrillo and Alaska Ranges. 15.8 Gt a −1 of calving flux comes from tidewater calving alone. This is quite extraordinary given that tidewater glaciers included in this estimate account for only 13% (ref. 47 ) of glacier area within the region examined. Given that lake and tidewater calving losses in Southeast Alaska are likely of comparable importance [2] , any changes in regional calving rates will have significant affects on total mass balance throughout the state. These data provide a first opportunity to partition mass loss for the region, which will help to constrain the evolution of SMB and calving into the future and consequently constrain SLR contributions from Alaska. Given a total annual mass budget of −47 Gt a −1 (estimated from GRACE [13] ), the annual net SMB (accumulation - ablation) would be ~−33 Gt a −1 or between −32 and −37 Gt a −1 . Given that Alaska is contributing 20% of the current SLR [1] , future changes in Alaska calving rates represent a significant SLR component that has few constraints on its evolution in a changing climate. Thus, it is of critical importance to begin reconcile mass change from calving, SMB models and GRACE in Alaska and to consider uncertainties in SMB and calving loss projections separately. These efforts will be key next steps towards reducing uncertainties in the rate of future mass loss in Alaska. Offset tracking Glacier surface velocities are derived using SAR offset tracking [31] , [33] with ALOS PALSAR Fine-Beam data (L-Band, HH Polarization, 46-day repeat). Repeat image pairs, acquired within one to two orbit intervals, are used to derive displacements. Raw (L0) data is processed to single-look complex (SLC) images using GAMMA software. Ground offsets are calculated from the slant-range SLCs using intensity cross-correlation optimization offset tracking [32] . SLCs are oversampled by a factor of two and all offsets with signal-to-noise ratios [32] below 5.0 are eliminated. A broad range of window sizes was tested; the chosen window size was 4590 pixels (nominally, 337 × 283 m). Wider windows tend to obtain more results, but are too large for use on small glaciers. Offsets are calculated at intervals of 20 × 40 pixels. Once offsets are calculated, they are geocoded, topographically corrected and corrected for image coregistration. These procedures require an elevation model. We choose the ASTER-GDEM 2.0 (ref. 48 ) because it extends throughout Alaska and is derived from comparatively recent data (1999–2011). Other elevation models are either dated (NED-DEM), limited to south of 60 ° latitude (SRTM-DEM), or unavailable at reasonable cost (SPOT-DEM). The ASTER-GDEM does have significant problems with artefacts and abrupt changes in elevation due to image saturation and changing surface heights over time, implications of these artefacts are discussed below. Offsets are geocoded using the GDEM and satellite geometry. Any offset estimate located on a DEM artefact will inherit a small error in that offset’s geo-location. Given that artefacts are relatively sparse and the final gridded data set is a smoothed interpolation from many offset estimates, the artefacts have little or no effect on the final map. Topographic correction is performed using concepts of radargrammetry [49] , where the corrected range offset, is a function of the measured offset, the elevation (obtained from the ASTER-GDEM), and the slave and master look angles. This approach is insensitive to errors in the GDEM, an error in the GDEM of 100 m, typically results in a range displacement error of <0.005 m per day. We correct for image coregistration by using the Randolph Glacier Inventory (RGI1.0) (ref. 47 ) and ASTER-GDEM to identify offsets that exist on stable ground (off-glacier and above 0 m elevation). The stable-ground offsets are modelled using a second-order polynomial function fit using an iterative least squares method. Residuals from each iterative fit are used to identify and eliminate outlying offsets and sequentially improve the model. Threshold residuals for exclusion from the fit are 3, 2.5 and 2 sigma values. The final polynomial is subtracted from all offsets to provide ice displacements on glaciers and uncertainty estimates off-glacier. Offset tracking creates many erroneous offset vectors, which are eliminated using a highly effective culling routine [50] . The routine filters vectors by comparing their orientation and magnitude to neighbouring vectors; it removes better than >99% of erroneous vectors and removes <0.1% false negatives. Each scene is also manually inspected for other problems, including removing any remaining offset vectors that are not pointing in the direction of flow or are anomalously high/low. A total of 624 frames are processed into 344 image pairs that encompass the Wrangell-St Elias Mountains, the Chugach, Kenai Peninsula, Alaska Range and Tordrillo Range. Then, custom software is used to manually identify which frames can best represent each glacier and then mosaic chosen offset vector fields from multiple frames. Temporal changes in flow velocity complicate the mosaicking process. The primary protocols for mosaicking include: avoid breaking up a glacier system between two different acquisition time periods to assure continuity for each glacier basin, for example, joining frames along ice divides or ridges rather than across a glacier. If protocol 1 is not possible given available data, frames are chosen that have the most comparable velocities at the seam. Overall, continuity within each glacier basin is prioritized above optimal spatial coverage. In total, 60 frames were chosen to produce the final maps. The dates of these image pairs are shown in Fig. 5 . The mosaicked vector field for each mountain range is interpolated onto 90 m UTM grids using a second-order polynomial regression with a search radius of 900 m. A minimum of six values must exist with at least 4 of 8 radial sectors surrounding a grid point to obtain an interpolated value. This method is effective at smoothing out minute differences in neighbouring vectors. As the mosaic contains data from different dates, and processing configurations, the pedigree of each individual vector is stored and interpolated onto the same UTM grid using nearest neighbour interpolation. Uncertainty estimation We provide an estimate of uncertainty by examining the distribution of offset vectors obtained on stable ground (off-glacier). Stable-ground offset vectors are obtained by masking each offset field with the RGI1.0 (ref. 47 ) data set and the ASTER-GDEM 2.0 (ref. 48 ) (eliminating ocean). Calculated offsets on stable ground have non-zero magnitudes due to erroneous correlation matches, errors in image coregistration and ambiguities in the location of the correlation peak. Erroneous correlation matches give the stable-ground offset fields a non-normal distribution (extremely large tails). Thus, we describe their distribution using robust, non-parametric statistics including median and normalized median absolute deviation (MADn, robust equivalent to s.d.) [51] . Estimated uncertainties for each image pair are displayed in Fig. 6 . Median values of off-glacier vectors (representing overall directional bias) are <0.003 m per day. Overall, the MADn values of off-glacier vectors averages 0.02 m per day in range and azimuth directions, in all cases the MADn is <0.06 m per day. 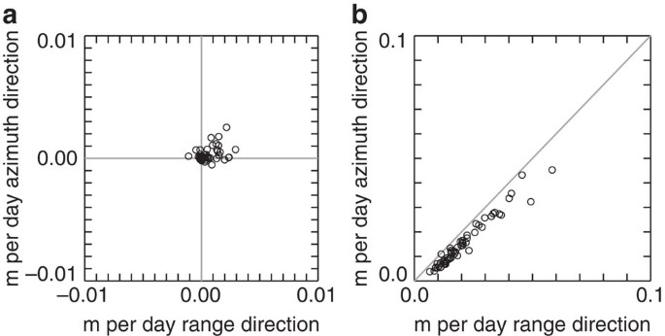Figure 6: Estimated uncertainties for all 60 image pairs. (a) Median values of all stable-ground offset vectors. (b) Mean normalized median absolute deviation (robust equivalent to s.d.) of all stable-ground offset vectors within each image pair, 1:1 line shown. Figure 6: Estimated uncertainties for all 60 image pairs. ( a ) Median values of all stable-ground offset vectors. ( b ) Mean normalized median absolute deviation (robust equivalent to s.d.) of all stable-ground offset vectors within each image pair, 1:1 line shown. Full size image Tidewater calving fluxes Tidewater calving fluxes are estimated across flux gates on 36 calving glaciers. Our flux estimates are subject to uncertainties in vertical and temporal velocity variability and large uncertainties in ice thickness. However, estimating uncertainty for calving fluxes in Alaska is difficult due to a lack of SMB, sliding velocity and ice thickness data. Therefore, we chose the simplest methods available and bracket our best estimate with high and low-end estimates. We use stationary flux gates, thus do not take into account retreating/advancing termini; nor do we account for mass lost through SMB between the flux gate and terminus. Seasonal variations in velocity are incorporated into our bracketed estimates as discussed below. Any missing data along each flux gate is interpolated using a spline interpolation that forces the velocity to zero at the glacier edge. Flow velocity perpendicular to the gate is integrated over the glacier width, yielding an areal surface flux ( Table 1 ). While effort was made to establish gates as close to termini as possible, our lack of data near some tidewater termini forces gates upstream. The median distance from each terminus to gate is 1.5 km or, on average, ~11% up the total glacier length. The mean gate elevation is 410 m and typical coastal Alaska equilibrium lines are at ~1,000 m. Thickness observations are unavailable at the flux gates, thus we obtain a crude thickness estimate using a well-established [52] square-root relationship between glacier length ( L ) and mean thickness ( H m ) (ref. 7 ), Where α m is a constant we assign a value of 2 (following Oerlemans [52] ). Given that our flux gates are roughly halfway between the equilibrium line and the terminus, we suggest that this mean glacier thickness is a reasonable value to use at each flux gate. Our best estimate assumes the mean glacier thickness from equation 2 and assumes the vertically integrated flow velocity is equivalent to the surface velocity (basal sliding usually dominates ice motion near tidewater termini as observed on Columbia Glacier [53] ). Our high-end estimate assumes the same thickness and vertical velocity profile as our best estimate, but also increases observed January–February velocities by 10% to account for seasonal velocity variability (a value based on seasonal variability at Hubbard Glacier [42] ). Our lowball estimate assumes 70% of the mean glacier thickness at the flux gate [52] and a vertically integrated flow velocity equivalent to 80% of the surface velocity (this is assuming perfect plasticity and no basal sliding [54] ). There are limited opportunities to validate these methods. Thickness observations from airborne low-frequency radar surveys on Seward and Bering Glaciers [55] conform well to mean thicknesses of 690 and 800 m derived from the method used here. However, mean thickness on Columbia Glacier [53] (determined from continuity modelling) is far lower than the mean thickness estimated by methods described here (145 and 440 m, respectively). Columbia is in a unique and rapid retreat [53] ; thus, it may not be a representative case. Nonetheless, this highlights the large uncertainties in glacier thickness estimates in Alaska. How to cite this article: Burgess, E. W. et al. Flow velocities of Alaskan glaciers. Nat. Commun. 4:2146 doi: 10.1038/ncomms3146 (2013).